Isotopic ordering in eggshells reflects body temperatures and suggests differing thermophysiology in two Cretaceous dinosaurs Our understanding of the evolutionary transitions leading to the modern endothermic state of birds and mammals is incomplete, partly because tools available to study the thermophysiology of extinct vertebrates are limited. Here we show that clumped isotope analysis of eggshells can be used to determine body temperatures of females during periods of ovulation. Late Cretaceous titanosaurid eggshells yield temperatures similar to large modern endotherms. In contrast, oviraptorid eggshells yield temperatures lower than most modern endotherms but ∼ 6 °C higher than co-occurring abiogenic carbonates, implying that this taxon did not have thermoregulation comparable to modern birds, but was able to elevate its body temperature above environmental temperatures. Therefore, we observe no strong evidence for end-member ectothermy or endothermy in the species examined. Body temperatures for these two species indicate that variable thermoregulation likely existed among the non-avian dinosaurs and that not all dinosaurs had body temperatures in the range of that seen in modern birds. Was non-avian dinosaur physiology similar to modern reptiles, which are ectotherms having body temperatures controlled by exchange of heat with the environment, or to modern endotherms such as mammals and birds that maintain high and stable body temperatures through metabolic heat production and strict thermoregulation [1] , [2] , [3] , [4] , [5] , [6] , [7] , [8] , [9] ? Endotherms are organisms that utilize internally generated heat to maintain their body at metabolically favourable temperatures. Ectotherms are organisms that have small or negligible internal heat production and rely on heat from the environment to reach metabolically favourable body temperatures. Alternatively, did some non-avian dinosaurs have physiological states intermediate between ectotherms and modern birds, conditions that have been termed basoendothermy or mesothermy [10] , [11] and have similarities to extant species such as lamnid sharks and monotremes [11] ? Basoendothermy has been defined as an endotherm with a body temperature of <35 °C (ref. 10 ). Mesotherms have been described as organisms that rely on metabolic heat to raise their body temperatures above ambient temperature, but that do not defend a thermal set point as do endotherms [11] . An intermediate thermophysiology has also been hypothesized for basal, pre-modern birds [12] , [13] . Body temperatures are not an unambiguous determinate of physiology as, for example, animals with low metabolic rate can have elevated body temperature as a result of high body mass and increased capacity to retain heat; a feature that is sometimes termed gigantothermy, as seen in extant species such as leatherback turtles [14] . Even within endotherms a wide range of physiological states exists, which can be reflected in body temperature [10] , [15] , [16] . Mesothermy in dinosaurs is supported by a recent theoretical study [11] and highlights that the debate on dinosaur thermophysiology is not a question of a simple ‘warm-blooded’ versus ‘cold-blooded’ dichotomy. Despite these complexities, body temperature determinations for extinct species place new constraints on physiology that were not previously possible, and allow us to test the predictions made by physiological models and growth rate analysis [17] , [18] . Here we constrain the body temperatures of extinct vertebrates from the analysis of proportions of multiply-substituted ( 13 C– 18 O-bearing; ‘clumped’) carbonate in fossil eggshells. The analysis of abundances of multiply-substituted, 13 C– 18 O-bearing molecules in carbonates is an emerging approach to constrain mineral formation temperatures [19] , [20] . Eggshells mineralize in the lower oviduct and so their isotopic composition should reflect body core temperatures of females during ovulation. In practice, the parameter measured is the Δ 47 value, which refers to the abundance of mass-47 CO 2 ( 13 C 18 O 16 O) in gas liberated by phosphoric acid digestion of carbonates compared with the abundance in reference gases of known isotopic composition CO 2 (refs 20 , 21 , 22 ). We have previously shown that Δ 47 measurements on CO 2 derived from carbonate moieties in biogenic phosphate minerals are correlated with the body temperature of the host animal [16] . Therefore, it is possible to reconstruct the body temperature of extinct vertebrates based on the measurement of isotopic ordering in fossil tooth enamel, but less reliably in the more readily diagenetically altered bone and tooth dentin [17] , [18] . CaCO 3 eggshells are another target for body temperature reconstructions and potentially allow determinations of body core temperatures in animals where enough well-preserved bioapatite material is not available. In addition, the stable isotope composition of eggshells may also record information on the environments in which an animal lived and their diet [23] , [24] , [25] . Clumped isotope data for modern eggshells Measurements were carried out on a suite of modern calcite and aragonite eggshells comprising specimens from 13 different bird species and 9 reptiles to establish the ability of Δ 47 measurements to distinguish between the body temperature of known endothermic and ectothermic animals. 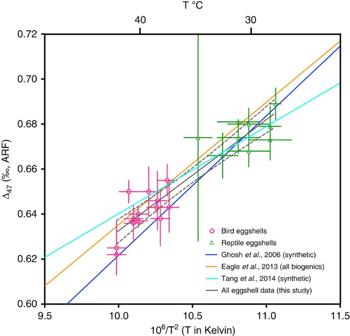Figure 1: Δ47measurements in modern eggshells. Data from modern bird and ectotherm eggshells are plotted against published inorganic calcite calibrations. Data are given inTable 1and temperature calibrations inSupplemental Note 2. By convention temperature is plotted as 106/T2(T in Kelvin) on thexaxis, but we indicate T in °C at the top of the plot. Linear regressions on the absolute reference frame were calculated as described previously28. Eggshell data and linear regression match more closely with the calibrations produced in the Caltech of Ghoshet al.19, and the Caltech all biogenics calibration of Eagleet al.26, than with that of Tanget al.41(Supplemental Note 2). The slope of the regression through eggshell data is described as: Δ47=0.0493±0.0043 (106T−2)+0.1393±0.0447. The data are presented in Table 1 and Fig. 1 show that this is clearly achievable, with Δ 47 -derived temperatures from bird and reptile eggshells mirroring known body temperature differences. In reptiles with small fluctuations in body temperature (for example, Galapagos tortoise), we also find that the average body temperature of the organism is accurately recorded by the eggshell. In organisms such as crocodilians that can exhibit more variability in body temperatures, we assumed ovulation occurred during the warm season given what is reported for survivorship of hatchlings in crocodilians and some other reptiles ( Supplementary Tables 1, 5 and 6 ). A caveat is that reptile body temperatures fluctuate daily and also vary depending on size and environment and thus the timing and temperature of eggshell mineralization may not be well constrained. Nevertheless, Δ 47 temperature determinations for reptiles are plausible average body temperatures for adults based on instrumental measurements ( Table 1 ; Supplementary Table 1 ; Fig. 1 ) and are clearly resolved from isotopic temperatures derived from bird eggshells ( Table 1 ). Eggshells from smaller bird species known to have elevated metabolic rates and body temperatures also yield higher Δ 47 -derived temperatures compared with large flightless birds that tend to have lower body temperatures ( Table 1 ). Table 1 Stable isotope data from modern eggshells. Data are compared with published calibrations in Fig. 1 . Full size table Figure 1: Δ 47 measurements in modern eggshells. Data from modern bird and ectotherm eggshells are plotted against published inorganic calcite calibrations. Data are given in Table 1 and temperature calibrations in Supplemental Note 2 . By convention temperature is plotted as 10 6 /T 2 (T in Kelvin) on the x axis, but we indicate T in °C at the top of the plot. Linear regressions on the absolute reference frame were calculated as described previously [28] . Eggshell data and linear regression match more closely with the calibrations produced in the Caltech of Ghosh et al . [19] , and the Caltech all biogenics calibration of Eagle et al . [26] , than with that of Tang et al . [41] ( Supplemental Note 2 ). The slope of the regression through eggshell data is described as: Δ 47 =0.0493±0.0043 (10 6 T −2 )+0.1393±0.0447. Full size image The application of a range of different temperature calibrations to modern eggshells produces results that match well with instrumental data on body temperatures. Using the calibration of Ghosh et al . [19] , the eggshell Δ 47 -derived temperatures ranging from 37 to 45 °C for different bird species are similar to directly determined bird body temperatures of 38–43 °C ( Table 1 ; Supplementary Note 2 ). Similar values of 36–45 °C are obtained using a calibration derived from a compilation of data generated from various biogenic carbonates in the Caltech lab ( Table 1 ; Supplementary Note 2 ) [26] , as well as other calibrations as described in the Supplementary Note 2 . We show in Fig. 1 and Supplementary Note 2 that the slopes of a regression through the eggshell data cannot be statistically distinguished from both the inorganic calcite calibration and biogenic data compilation generated at Caltech [19] , [26] . For completeness, Δ 47 -based temperatures are estimated using four different calibrations ( Supplementary Tables 1–3 ), although in the main text and figures we favour application of the Caltech biogenic calibration because it is based on the largest data set and therefore has lower uncertainty [26] . While it would be possible to use the eggshell-specific calibration, it is less data-rich and has uncertainties associated with not knowing precisely the expected body temperatures at which ectotherms mineralize their eggshells, and as a result is less constrained than the Caltech biogenic calibration ( Supplementary Note 2 ). Preservation of fossil eggshells Fossil eggshells likely have a higher potential for preservation than dentin and bone; high porosity, small crystal sizes and high protein and water contents (c. 50%) in the latter two materials/tissues tend to lead to massive recrystallization and isotopic resetting during fossilization [27] . This contrasts with the rigid CaCO 3 -dominated eggshells that many organisms produce. For example, chicken eggshells are 95–97% CaCO 3 and therefore comprise much lower levels of organic matter than bone and dentin [28] . As geochemical preservation represents a key uncertainty in our analysis, here we have taken the approach of extensively characterizing each specimen using a hierarchy of approaches. First, a comparative analysis of the stable isotope and trace-element composition of the eggshell and associated carbonates, including diagenetically altered bone and authigenically formed spar calcite, is used with the reasoning that unaltered primary eggshells will usually be different in composition from coexisiting carbonates from other origins ( Fig. 2 ; Supplementary Figs 4–6 ). Second, we examined thin sections of specimens using transmitted light microscopy and eggshell fragments using scanning electron microscopy to confirm the retention of primary growth textures and to look for diagenetic features ( Fig. 3 ; Supplementary Note 3 ; Supplementary Figs 1–3 ). We also carried out electron backscatter diffraction (EBSD) analysis to examine specimens for changes in calcite crystallographic orientation associated with eggshell recrystallization ( Figs 4 , 5 ; Supplementary Fig. 7 ). 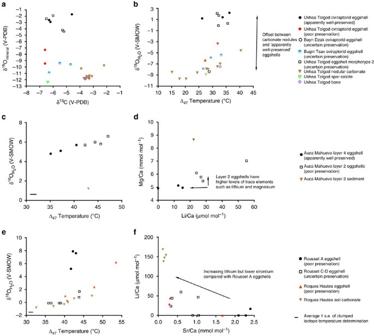Figure 2: Examples of isotopic and trace-element data used to assess preservation. Supplementary Tables 1–3contain raw data. Additional data plots are given inSupplementary Figs 4–6. (a,b) Data from Mongolian samples. (b) Illustration of the large offset between the calculated waterδ18O for three apparently well-preserved eggshells from Ukhaa Tolgod, and nodular and spar carbonates recovered from the same strata. Two other eggshells from Ukhaa Tolgod do not show this offset and so were considered of poor preservation. Detailed description of the other Mongolian eggshell types and their preservation can be found in the main text andSupplementary Notes 1 and 3, but all were considered of uncertain preservation due to either petrographic analysis or the fact that they were from a different site and so the comparison between them and other carbonate phases was not possible. (c,d) Data from Auca Mahuevo samples. Δ47temperatures are noticeably higher for layer-2 specimens, compared with layer-4 specimens; layer-2 specimens are also higher in contents of elements such as lithium and magnesium which, in addition to petrographic and scanning electron microscopy analysis, lead to us considering layer-4 specimens to be better preserved. (e,f) Data from Provence Basin samples. Eggshells from the Rousset locality, stratigraphic layer A, are notably distinct in both carbonateδ18O (not shown) and calculatedδ18O of mineral formation water. Rousset A eggshells are also comparatively enriched in strontium, but lower in lithium compared with eggshells from other stratigraphic layers and eggshells and soil carbonate nodules from the nearby Roques Hautes site. Rousset A are distinct geochemically and eggshells were found to be most altered by EBSD analysis (Fig. 5;Supplementary Fig. 7). Figure 2: Examples of isotopic and trace-element data used to assess preservation. Supplementary Tables 1–3 contain raw data. Additional data plots are given in Supplementary Figs 4–6 . ( a , b ) Data from Mongolian samples. ( b ) Illustration of the large offset between the calculated water δ 18 O for three apparently well-preserved eggshells from Ukhaa Tolgod, and nodular and spar carbonates recovered from the same strata. Two other eggshells from Ukhaa Tolgod do not show this offset and so were considered of poor preservation. Detailed description of the other Mongolian eggshell types and their preservation can be found in the main text and Supplementary Notes 1 and 3 , but all were considered of uncertain preservation due to either petrographic analysis or the fact that they were from a different site and so the comparison between them and other carbonate phases was not possible. ( c , d ) Data from Auca Mahuevo samples. Δ 47 temperatures are noticeably higher for layer-2 specimens, compared with layer-4 specimens; layer-2 specimens are also higher in contents of elements such as lithium and magnesium which, in addition to petrographic and scanning electron microscopy analysis, lead to us considering layer-4 specimens to be better preserved. ( e , f ) Data from Provence Basin samples. Eggshells from the Rousset locality, stratigraphic layer A, are notably distinct in both carbonate δ 18 O (not shown) and calculated δ 18 O of mineral formation water. Rousset A eggshells are also comparatively enriched in strontium, but lower in lithium compared with eggshells from other stratigraphic layers and eggshells and soil carbonate nodules from the nearby Roques Hautes site. Rousset A are distinct geochemically and eggshells were found to be most altered by EBSD analysis ( Fig. 5 ; Supplementary Fig. 7 ). 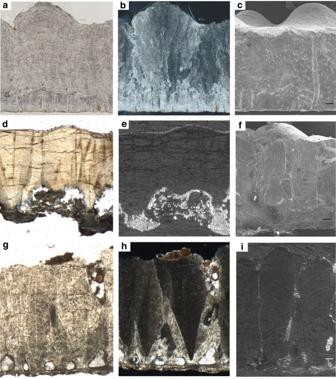Figure 3: Petrographic and scanning electron microscopy characterization of dinosaur eggshells. Representative images are shown. (a,b) Light and polarized light images of a thin section of an apparently well-preserved Oviraptorid eggshell from Ukhaa Tolgod, Mongolia. (c) scanning electron microscopy (SEM) image of a cross-section of the eggshell. Pores such as the one indicated are small and rare compared with Titanosaurid eggshells. As pores are often foci for dissolution and secondary mineral formation, this may be a reason for the relatively good preservation of the Oviraptorid eggshells. (d,e) Light and cathodoluminescence images of an Auca Mahuevo titanosaur layer-2 eggshell showing localized areas of secondary carbonate on the upper and lower surface.(f) SEM image of an Auca Mahuevo layer-4 eggshell. Importantly, energy-dispersive X-ray analysis (EDS) of material infilling Auca Mahuevo eggshell pores found that it was silica-rich clay rather than secondary calcite (Supplementary Note 3). (g–i) Light, polarized light and cathodoluminescence images of typical eggshells from the Rousset site in the Provence Basin. Secondary carbonate is often found on the exterior surfaces and infilling the pores of eggshells from this site, as shown in the cathodoluminescence image. In some cases, Rousset eggshells were found to have a strong cathodoluminescence signal from within the main eggshell structure, a clear indication of alteration (Supplementary Fig. 3). Scale bar (c)∼100 mm); (f,i) 200 mm. More examples of this type of analysis and more in-depth interpretations can be found in theSupplementary Note 3andSupplementary Figs 1–7. Full size image Figure 3: Petrographic and scanning electron microscopy characterization of dinosaur eggshells. Representative images are shown. ( a , b ) Light and polarized light images of a thin section of an apparently well-preserved Oviraptorid eggshell from Ukhaa Tolgod, Mongolia. ( c ) scanning electron microscopy (SEM) image of a cross-section of the eggshell. Pores such as the one indicated are small and rare compared with Titanosaurid eggshells. As pores are often foci for dissolution and secondary mineral formation, this may be a reason for the relatively good preservation of the Oviraptorid eggshells. ( d , e ) Light and cathodoluminescence images of an Auca Mahuevo titanosaur layer-2 eggshell showing localized areas of secondary carbonate on the upper and lower surface. ( f ) SEM image of an Auca Mahuevo layer-4 eggshell. Importantly, energy-dispersive X-ray analysis (EDS) of material infilling Auca Mahuevo eggshell pores found that it was silica-rich clay rather than secondary calcite ( Supplementary Note 3 ). ( g – i ) Light, polarized light and cathodoluminescence images of typical eggshells from the Rousset site in the Provence Basin. Secondary carbonate is often found on the exterior surfaces and infilling the pores of eggshells from this site, as shown in the cathodoluminescence image. In some cases, Rousset eggshells were found to have a strong cathodoluminescence signal from within the main eggshell structure, a clear indication of alteration ( Supplementary Fig. 3 ). Scale bar ( c ) ∼ 100 mm); ( f , i ) 200 mm. More examples of this type of analysis and more in-depth interpretations can be found in the Supplementary Note 3 and Supplementary Figs 1–7 . 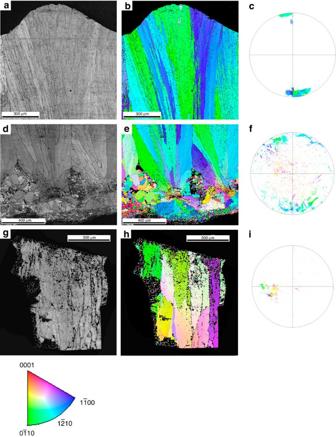Figure 4: EBSD analysis of Auca Mahuevo eggshells. Images are representative of multiple specimens examined. (a,d,g) Grayscale diffraction maps in which lighter regions represent areas where greater diffraction is observed. (b,e,h) Colours represent different crystallographic planes of calcite, as shown in the colour-coded legend given in the bottom of the figure. (c,f,i) The corresponding pole figures of the planes projected on the {0001} plane of calcite. (a–c) Analysis of the prismatic layer (exterior portion, or palisade layer) of a titanosaur eggshell from Auca Mahuevo layer 4. This section of the eggshell exhibits excellent preservation on EBSD analysis, with the alternation {0–110} and {1–100} planes of calcite in the cross-section and thecaxis parallel to the elongation of calcite crystals and perpendicular to the shell exterior, and seen in some modern avian eggshells42and consistent with previous studies on titanosaur eggshells43. (d–f) Mammilla (inner) layers of the same eggshell, also exhibiting excellent preservation in the regions where calcite crystals fan out from the cones and thecaxis parallel to their elongation, but have a less constrained distribution of poles as shown in the pole figure (f). Areas between the cones were likely originally organic rich, but are now partially replaced by secondary calcite crystals (isolated orange–yellow–red poles inf). A similar feature can often be observed in both layer-2 and layer-4 Auca Mahuevo eggshells by cathodoluminescence, for exampleFig. 3e. As described in the Methods, this area of secondary calcite on the interior surface is likely removed by drilling during the preparation stage. (g–i) Auca Maheuvo layer-2 eggshell that is heavily recrystallized. Each calcite crystal has a different orientation and without a preferred orientation of thecaxis of calcite, indicative of recrystallization. The diffraction map shows regular edges of calcite crystals, defining prisms, which would suggest that the recrystallization is due to a closed-system replacement rather than open-system recrystallization involving dissolution and precipitation of secondary calcite. Full size image Figure 4: EBSD analysis of Auca Mahuevo eggshells. Images are representative of multiple specimens examined. ( a , d , g ) Grayscale diffraction maps in which lighter regions represent areas where greater diffraction is observed. ( b , e , h ) Colours represent different crystallographic planes of calcite, as shown in the colour-coded legend given in the bottom of the figure. ( c , f , i ) The corresponding pole figures of the planes projected on the {0001} plane of calcite. ( a – c ) Analysis of the prismatic layer (exterior portion, or palisade layer) of a titanosaur eggshell from Auca Mahuevo layer 4. This section of the eggshell exhibits excellent preservation on EBSD analysis, with the alternation {0–110} and {1–100} planes of calcite in the cross-section and the c axis parallel to the elongation of calcite crystals and perpendicular to the shell exterior, and seen in some modern avian eggshells [42] and consistent with previous studies on titanosaur eggshells [43] . ( d – f ) Mammilla (inner) layers of the same eggshell, also exhibiting excellent preservation in the regions where calcite crystals fan out from the cones and the c axis parallel to their elongation, but have a less constrained distribution of poles as shown in the pole figure ( f ). Areas between the cones were likely originally organic rich, but are now partially replaced by secondary calcite crystals (isolated orange–yellow–red poles in f ). A similar feature can often be observed in both layer-2 and layer-4 Auca Mahuevo eggshells by cathodoluminescence, for example Fig. 3e . As described in the Methods, this area of secondary calcite on the interior surface is likely removed by drilling during the preparation stage. ( g – i ) Auca Maheuvo layer-2 eggshell that is heavily recrystallized. Each calcite crystal has a different orientation and without a preferred orientation of the c axis of calcite, indicative of recrystallization. The diffraction map shows regular edges of calcite crystals, defining prisms, which would suggest that the recrystallization is due to a closed-system replacement rather than open-system recrystallization involving dissolution and precipitation of secondary calcite. 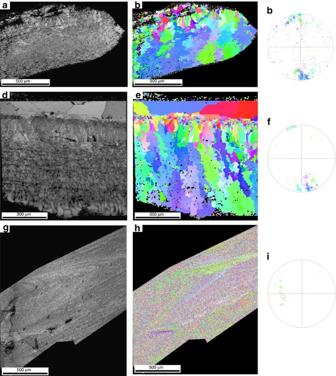Figure 5: EBSD analysis of Mongolian and French eggshells. Images are representative of multiple specimens examined. Colour coding is as described inFig. 4. (a–c,d–f) Two different individual Mongolian Oviraptorid eggshells, respectively. Both eggshells show an overall good preservation, with no evidence for recrystallization and calcite crystals displaying a preferred crystallographic orientation of thecaxis perpendicular to the shell exterior, as shown in pole figures. In this respect, data are similar to Auca Mahuevo layer-4 eggshells inFig. 4. There are some indications of deformation of calcite crystals, possibly due to eggshells being compressed on burial, as indicated discontinuity and deformation of crystal boundaries as seen in diffraction maps and a larger spreading of poles on the projection of the {0001} plane of calcite than typically observed in modern eggshells. For comparison, the bottom panels (g–i) show data from a Rousset level-A eggshell that is completely altered and recrystallized, with none of the original microstructure typical of eggshells observed. Instead, the eggshell has been replaced by microcrystalline calcite with low diffraction, and the pole figure (i) shows the absence of biological control over crystallographic orientation. Full size image Figure 5: EBSD analysis of Mongolian and French eggshells. Images are representative of multiple specimens examined. Colour coding is as described in Fig. 4 . ( a – c , d – f ) Two different individual Mongolian Oviraptorid eggshells, respectively. Both eggshells show an overall good preservation, with no evidence for recrystallization and calcite crystals displaying a preferred crystallographic orientation of the c axis perpendicular to the shell exterior, as shown in pole figures. In this respect, data are similar to Auca Mahuevo layer-4 eggshells in Fig. 4 . There are some indications of deformation of calcite crystals, possibly due to eggshells being compressed on burial, as indicated discontinuity and deformation of crystal boundaries as seen in diffraction maps and a larger spreading of poles on the projection of the {0001} plane of calcite than typically observed in modern eggshells. For comparison, the bottom panels ( g – i ) show data from a Rousset level-A eggshell that is completely altered and recrystallized, with none of the original microstructure typical of eggshells observed. Instead, the eggshell has been replaced by microcrystalline calcite with low diffraction, and the pole figure ( i ) shows the absence of biological control over crystallographic orientation. Full size image On the basis of these analyses, we found specimens exhibited a range of preservation states. We characterized specimens to be ‘apparently well preserved’ if we had no reason to reject them as diagenetically altered, ‘moderately preserved’ if geochemical evidence suggested they are well preserved but petrographic analysis suggested some evidence of alteration, ‘poorly preserved’ when clear evidence of alteration existed by any criteria and, finally, ‘of uncertain preservation’ where there was not enough information to judge, for example, because it was not possible to compare diagenetic phases and potentially preserved fossil material due to the availability of samples ( Table 2 ; Supplementary Note 3 ). Table 2 Stable isotope data from Cretaceous eggshells and associated phases. Full size table The fossil eggshells that we examined were collected from Upper Cretaceous formations from three main regions: (1) the Campanian and Maastrichtian Djadokhta (Ukhaa Tolgod and Bayn Dzak sites) and Nemegt (Bugin Tsav site) Formations, Nemegt Basin, Mongolia [29] ; (2) the Upper Cretaceous Anacleto Formation at Auca Mahuevo, Neuquén Province, Argentina [30] ; (3) the Maastrichtian Rousset and Roques Hautes sections, Provence Basin, France [31] , [32] . Eggshells from the Late Cretaceous of Montana, Spain, Rio Negro in Argentina and a second eggshell morphotype from the Nemegt Basin of Mongolia were less constrained taxonomically and so are not discussed in detail here but are described in Supplementary Note 3 . The taxonomic identity of the oviraptorid theropod and titanosaurid sauropod eggshells from Mongolia and Argentina, respectively, was determined on the basis of in situ embryos [30] , [33] , whereas the taxonomic identity of French eggshells is inferred based on eggshell morphology and proximity to other fossil remains in the same strata [31] . Therefore, the eggshells from the Provence basin are designated ‘putative titanosaurid’. Oviraptorid eggshell specimens from the Djadokhta and Nemegt Formations showed generally good preservation based on petrographic observations, with most confirmed oviraptorid eggshells showing little or no evidence for alteration by inspection of thin sections or eggshell fragments ( Supplementary Note 3 ; Supplementary Fig. 1 ). EBSD analysis showed no evidence for recrystallization of these specimens and also showed the preferred crystallographic orientation of the calcite c axis is present, but it did suggest some deformation of calcite crystals, possibly due to compression of the eggshells on burial ( Fig. 5 ). It is not clearly known what impact this type of crystal deformation could have on clumped isotope signatures. Although this feature is widespread in the oviraptorid eggshells examined here, measured clumped isotope values do not show evidence for extensive bond reordering, which would be expected to yield significantly lower Δ 47 values than would be compatible with plausible body temperatures and the values measured ( Table 2 ). Therefore, we continued to consider these specimens apparently well preserved, with the caveat that the impact of compression is not fully understood. The majority of eggshells from the Djadokhta Formation at Ukhaa Tolgod are geochemically distinct from abiogenic nodular carbonates, bone and spar calcites recovered from the same site, indicating that pervasive diagenesis of carbonates had not occurred. Two eggshells from Ukhaa Tolgod were considered poorly preserved, as their isotopic composition approached that of known diagenetic phases such as sparry calcites and altered bone ( Supplementary Table 3 ; Supplementary Fig. 4 ). Ukhaa Tolgod morphotype 2 eggshells were considered of uncertain preservation, as petrographic analysis suggested that they had areas of dissolution in the main eggshell structure that was much more extensive than in the oviraptorid specimens from the same site, but geochemically they were also distinct from diagenetic phases ( Fig. 2 ; Supplementary Fig. 1 ; Supplementary Note 3 ). Four specimens from the Bayn Dzak and Bugin Tsav localities were considered of uncertain preservation as they had similar isotopic composition as diagenetic phases from Ukhaa Tolgod, although we note that, as they are from a different locality, this comparison may be less instructive. It is possible that primary and diagenetic carbonate phases could be fortuitously similar to one another in composition, and therefore our approach to excluding data is a conservative one. Auca Mahuevo titanosaurid specimens from different stratigraphic horizons are variably preserved based on geochemical, petrographic and EBSD analysis ( Figs 2 , 3 , 4 ; Supplementary Note 3 ; Supplementary Figs 2 and 5 ). Notably, EBSD analysis revealed complete recrystallization of some layer-2 eggshells and good preservation of layer-4 eggshells ( Fig. 5 ). Layer-4 eggshells are therefore considered apparently well preserved by our criteria, but layer-2 specimens of poor preservation. Rousset level-A eggshells are geochemically distinct from soil carbonates and the other eggshells from this basin, indicating differential preservation ( Supplementary Figs 3 and 6 ). In this case EBSD analysis was instructive, as Rousset level-A eggshells were found to be completely recrystallized with little of the normal biological control of crystallographic orientation observable ( Fig. 5 ; Supplementary Fig. 7 ). Eggshell specimens from Roques Hautes in the Provence Basin are considered to be of poor preservation as microcharacterization showed evidence for secondary carbonate infilling of pore canals, and geochemically the eggshells had similar composition to contemporaneous soil carbonate nodules ( Fig. 2 ; Supplementary Figs 3 and 6 ). Rousset B–D eggshells also show overlap in isotopic composition with Roques Hautes soil carbonates ( Fig. 2 ). Petrographic and EBSD analysis of Rousset B–D eggshells yielded a mixed picture with some eggshells showing clear evidence of alteration, while others looking well preserved ( Fig. 3 ; Supplementary Figs 3 and 7 ). This is an indication that eggshells from these strata are variably preserved and may even have areas of better and worse preservation within the same individual specimen. For this reason, we considered these specimens of uncertain preservation. One clear finding from our study is that eggshell specimens from different stratigraphic layers of the same formation can show very different states of preservation, and that variability can also exist within a stratigraphic layer. Full justifications of our assessment of the preservation of each specimen including geochemical data and representative petrographic and scanning electron microscopy images can be found in Supplementary Note 2 . Body temperature determinations from fossil eggshells The apparently well-preserved Mongolian oviraptorid eggshells yield Δ 47 -derived temperatures of 31.9±2.9 °C (2 s.e. ), and the Auca Mahuevo layer-4 titanosaur eggshells yield temperatures of 37.6±1.9 °C ( Table 2 ), supporting differing thermoregulation between these species. Rousset level-B–D specimens yielded Δ 47 temperatures of 39.6±1.4 °C ( Table 2 ) and so also supporting high body temperatures for some dinosaurs, although these data should be regarded as less reliable than data from Auca Mahuevo layer-4. Nevertheless, our confidence in the finding of relatively high body temperatures in sauropod dinosaurs is increased by their close agreement with previous results of carbonate-clumped isotope thermometry of sauropod teeth [18] . Geochemical data for soil carbonates, poorly preserved eggshells and known diagenetic phases (altered bone and spar calcites) are also presented for comparison ( Fig. 2 ; Table 2 ; Supplementary Figs 1–6 ). We have shown that when applied to eggshells, carbonate ‘clumped isotope’ paleothermometry can be used to reconstruct body temperatures. While uncertainties regarding preservation of clumped isotopic signals in fossil eggshells remain, through a hierarchy of approaches we identify a number of dinosaur eggshell specimens that we have no reason to reject as being altered. Below we discuss the compatibility of Δ 47 temperatures from the apparently well-preserved specimens with other data and with previous inferences on the nature of non-avian dinosaur physiology. The comparison between oviraptorid eggshell Δ 47 temperatures and those measured from contemporaneous nodular carbonates recovered from the same strata is important (31.9 versus 26.3 °C respectively; Table 2 ). Δ 47 temperatures from nodular paleosol carbonates have been shown to reflect warm month average temperatures [34] . Therefore, the ∼ 6 °C higher temperatures derived from eggshells compared with nodular carbonates at Uhkaa Tolgod likely indicates that the oviraptorid dinosaurs were able to elevate body temperatures above environmental temperatures even when considering the warmest time of year. This interpretation would be supported even if partial alteration of 13 C– 18 O signatures had influenced the absolute value of the oviraptorid body temperature determinations, because measurements on spar calcite and nodular carbonates from this site suggests that if diagenesis of oviraptorid eggshells had occurred it would likely have driven Δ 47 temperatures towards colder values, not hotter ( Table 2 ). High body temperatures for large sauropod dinosaurs found here and in a previous study of sauropod teeth [18] could be a result of endothermy comparable to large extant mammals and birds, but could also reflect gigantothermy. Our finding in this study of lower temperatures in oviraptorid eggshells extends the range of inferred body temperatures in dinosaurs. Our oviraptorid data coupled with the sauropod data suggest that non-avian dinosaurs could be significantly variable in their thermoregulation and did all not have uniformly high ( ∼ 36–43 °C) body temperatures as modern birds do ( Fig. 6 ). These data are potentially consistent with a relationship between dinosaur body mass and body temperature, but if such a relationship exists it would need more data to accurately constrain. Regardless, the fact that oviraptorid dinosaurs apparently could maintain body temperatures above those of the environment suggests that either they were ectotherms having thermoregulatory behaviours or other adaptations such as insulation, or that they had a metabolism and thermal physiology intermediate between ectotherms and extant birds ( Fig. 4 ). Additional evidence supporting an intermediate physiology includes analysis of growth rates and sexual maturation in oviraptorids, which showed that sexual maturation occurred well before adult size was reached—a feature that is shared with reptiles and basal pre-modern birds [12] , [13] , but not extant birds [35] . In addition, recent theoretical work based on growth rate analysis has provided evidence for mesothermy in a range of non-avian dinosaurs [11] . 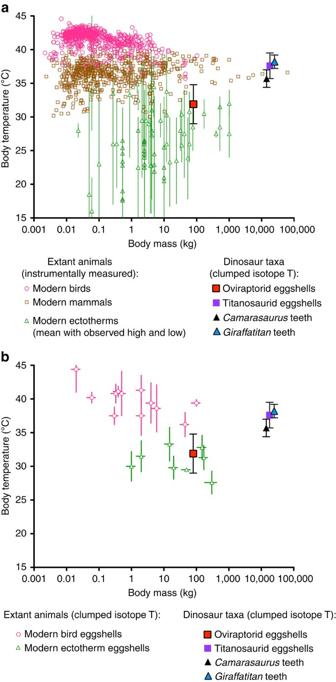Figure 6: Isotope-derived dinosaur body temperatures in context with modern species data. (a) Isotopic dinosaur body temperature determinations plotted versus compilations of modern mammal, bird and ectotherm body temperatures and body masses (Supplementary Tables 5 and 6). Error bars on dinosaur body temperature estimates represent two s.e. Clumped isotope-based temperature determinations from teeth of JurassicCamarasaurusandGiraffatitan18plotted alongside determinations from titanosaurid eggshells from Auca Mahuevo, Argentina, and oviraptorid eggshells from Ukhaa Tolgod, Mongolia. Modern ectotherm data points are calculated mean values with measured upper and lower limits indicated by grey bars (Supplementary Table 6). Clumped isotope estimates of oviraptorid dinosaur body temperatures are lower than all modern birds and most modern mammals, but are comparable to a minority of modern mammals. Isotopic estimates of oviraptorid dinosaur body temperatures are higher than most calculated mean ectotherm body temperatures but fall within the range exhibited by many ectotherms, including those of similar mass. Sauropod dinosaur (that is, titanosaurid,Camarasaurus,Giraffatitan) body temperatures are higher than the mean and range exhibited by the majority modern reptiles in this compilation. (b) Clumped isotope-based temperature determinations for both modern eggshells and dinosaur fossils. Monitor lizard eggshell isotope data with high error is excluded from this figure. Figure 6: Isotope-derived dinosaur body temperatures in context with modern species data. ( a ) Isotopic dinosaur body temperature determinations plotted versus compilations of modern mammal, bird and ectotherm body temperatures and body masses ( Supplementary Tables 5 and 6 ). Error bars on dinosaur body temperature estimates represent two s.e. Clumped isotope-based temperature determinations from teeth of Jurassic Camarasaurus and Giraffatitan [18] plotted alongside determinations from titanosaurid eggshells from Auca Mahuevo, Argentina, and oviraptorid eggshells from Ukhaa Tolgod, Mongolia. Modern ectotherm data points are calculated mean values with measured upper and lower limits indicated by grey bars ( Supplementary Table 6 ). Clumped isotope estimates of oviraptorid dinosaur body temperatures are lower than all modern birds and most modern mammals, but are comparable to a minority of modern mammals. Isotopic estimates of oviraptorid dinosaur body temperatures are higher than most calculated mean ectotherm body temperatures but fall within the range exhibited by many ectotherms, including those of similar mass. Sauropod dinosaur (that is, titanosaurid, Camarasaurus , Giraffatitan ) body temperatures are higher than the mean and range exhibited by the majority modern reptiles in this compilation. ( b ) Clumped isotope-based temperature determinations for both modern eggshells and dinosaur fossils. Monitor lizard eggshell isotope data with high error is excluded from this figure. Full size image The results presented here are striking given what is considered a close relationship between Oviraptoridae and birds, suggesting the endothermy of modern birds was not present in at least this one species of non-avian theropod dinosaurs. This proposition is also congruent with interpretations based on histological analysis of pre-modern birds, where it is proposed that basal birds were also not fully endothermic in comparison with extant species and that full endothermic homoeothermy evolved later and after the evolution of feathers and flight [12] , [13] . Our novel data therefore provide independent evidence to support inferences from histology and physiological modelling that some dinosaurs were not fully endothermic as are modern birds. Although we cannot extrapolate how representative oviraptorid body temperatures are of theropods, or non-avian dinosaurs more broadly, at least in this one case our data combined with published growth rate analyses [35] are consistent with a reduced form of endothermy described elsewhere as ‘mesothermy’ or ‘basoendothermy’ [10] , [11] . Specimens Modern eggshell specimens were obtained from a number of different sources including the Los Angeles Zoo, the San Francisco Zoo, the Zurich Zoo, the Western Foundation of Vertebrate Zoology, the South Carolina Zoo, private farms and collections. Full details on sources can be found in Supplementary Note 1 . The principle localities of fossil material were the Cretaceous strata in the Nemegt Basin, Mongolia, Auca Mahuevo in Neuquén Province, Argentina and the Provence Basin in France. Fossil specimens were sourced from the American Natural History Museum in New York, the Natural History Museum of Los Angeles County and the Goldfuß-Museum in Bonn. Full details regarding the specimens and their geological setting can be found in Supplementary Note 1 . Stable isotope analysis As described in more detail below, even eggshells with apparently good preservation as revealed by petrographic examination frequently show some evidence for dissolution and replacement on their outer surfaces and around pore canal openings. Therefore, we routinely drilled off and discarded the outer surface of eggshell specimens. After this initial preparation, a section of eggshell was broken off and powdered with a pestle and mortar. Where possible, soil carbonate nodules, spar calcites and bone samples were also drilled out and analysed but were not subject to any sample pretreatment. A total of 8–10 mg of carbonate and 120 mg of phosphate was reacted for 20 min in a common phosphoric acid bath heated to 90 °C. Product CO 2 was then purified using the automated online system, described previously [34] . This automated purification system includes passing sample gas through a Porapak Q 120/80 mesh GC column at −20 °C to remove potential organic contaminants and silver wool (Sigma-Aldrich) to remove sulfur compounds. Purified sample gases were then analysed on a Thermo Scientific MAT253 dual-inlet gas source mass spectrometer at Caltech using a published configuration and methods [22] . Reference gases of different compositions that had been heated to 1,000 °C to approximate a stochastic ‘random’ distribution of isotopes were also analysed to provide a reference frame for sample Δ 47 values. Carbonate standards were analysed every 5–6 analyses. The average external reproducibility (one s.e.) of Δ 47 measurements presented here is 0.008‰. Supplementary Table 7 contains the heated gas slope and intercepts, and secondary transfer function slope and intercepts. Data processing and calculation Δ 47 Values are defined as follows: Where R i represents mass i /mass 44 and R * represents the abundance of isotopologues in a sample with the same bulk isotopic composition, but that conforms to a random (stochastic) distribution [24] . For this study, an acid digestion correction of 0.081‰ was applied as described previously [34] . The vast majority of data for this study was collected before the proposition of an ‘absolute reference frame’ (ARF) for clumped isotope studies of CO 2 based on the analysis of water-equilibrated CO 2 gases [20] . Therefore, we converted Δ 47 values into the ARF by applying a secondary transfer function described previously [20] , which uses an accepted value of the standards NBS-19 and Caltech Carrara Marble of 0.392‰, and TV03 of 0.713‰. For calcite δ 18 O calculations, an acid digestion fractionation factor of 1.007954 was used [35] . For aragonite δ 18 O calculations an acid digestion fractionation factor of 1.00854126 was used, calculated by extrapolation from a published calibration [37] . Temperatures estimated using sample Δ 47 values were used to calculate the δ 18 O of water from which the mineral precipitated using paired measurements of carbonate δ 18 O and the following published equation [38] . For turtle and tortoise eggshells made of aragonite, the following equation was used from Kim et al . (2007) [37] : Propagated errors in water δ 18 O calculations were calculated as follows: Where E is one s.e. To derive the E 2 T term for calculating the propagated error in δ 18 O, the uncertainty in the Δ 47 -derived temperature is converted into a per mil value using the appropriate equation. Elemental analysis and microscopy Element to calcium ratios (Mg/Ca, Sr/Ca, Mn/Ca, Fe/Ca and Li/Ca) on splits of the same powders analysed for stable isotopes were determined on a Jobin-Yvon Ultima-C Inductively Coupled Atomic Emission Spectrometer [39] . Eggshell fragments were also inspected for diagenetic features and by scanning electron microscopy and energy-dispersive spectroscopy using a Tescan Vega-3 XMU variable-pressure scanning electron microscope. Petrographic analysis of thin sections of eggshells was carried out by polarized light and cathodoluminescence. EBSD analysis was carried out using a Hikari camera mounted on a TESCAN LYRA FIB-FESEM (field emission scanning electron microscope) [40] . Also see Supplementary Note 3 and Supplementary Figs 1–7 for the results and discussion of this analysis. Modern taxa body temperature data Stable isotope data for modern eggshells are in Table 1 and Supplementary Tables 1 and 2 . Modern taxa body temperature data and associated references are given in Table 1 , and Supplementary Tables 5 and 6 . Expected temperatures for birds have an uncertainty of ±0.2–0.5 °C associated with data loggers used; if no error was reported in the study, then we assumed a conservative value for the temperature uncertainty. In reptiles with small fluctuations in body temperature (for example, Galapagos tortoise), the average body temperature is accurately recorded by the eggshell. In organisms such as crocodilians that are from environments with more variability in body temperatures, we used warm season temperatures given what is reported for survivorship in crocodilians and some other reptiles: extremely high mortality rates in hatchlings of up to 100% are reported when environmental or incubation temperatures are below 27 °C. Thus crocodilian body temperatures associated with eggshell formation are likely to reflect warm season conditions and not growth during winter in environments with moderate seasonality. In Supplementary Note 2 we discuss whether published calibrations reproduce these temperatures, and then discuss a Δ 47 -temperature calibration produced using the modern eggshell data. Δ 47 -Temperature calibrations The Δ 47 -temperature calibrations utilized in the main text are the initial inorganic calcite calibration produced in the Caltech lab converted to the absolute reference frame (Δ 47 =0.0636 (10 6 T −2 )–0.0047) [19] , [20] and the ‘all biogenic materials’ compilation of data from the Caltech lab (Δ 47 =0.0559 (10 6 T −2 )+0.0708) [26] . Temperature is in Kelvin (K). A growing number of alternative calibrations have been published, many of which we find do not yield plausible Δ 47 -derived body temperatures from our eggshell data, as described in more detail in Supplementary Note 2 . Therefore, while Δ 47 calibrations remain largely empirical, the eggshells studied here appear to be equivalent to the majority of biogenic material studied to date in the Caltech lab ( Fig. 1 ) and suggest that alternative calibrations with shallower slopes ( Supplementary Note 2 ) may not apply to all biogenic materials analysed at Caltech with the same experimental set-up and during similar analytical time periods (2008–2015). How to cite this article: Eagle, R. A. et al . Isotopic ordering in eggshells reflects body temperatures and suggests differing thermophysiology in two Cretaceous dinosaurs. Nat. Commun. 6:8296 doi: 10.1038/ncomms9296 (2015).